Impedance sensing device enables early detection of pressure ulcersin vivo When pressure is applied to a localized area of the body for an extended time, the resulting loss of blood flow and subsequent reperfusion to the tissue causes cell death and a pressure ulcer develops. Preventing pressure ulcers is challenging because the combination of pressure and time that results in tissue damage varies widely between patients, and the underlying damage is often severe by the time a surface wound becomes visible. Currently, no method exists to detect early tissue damage and enable intervention. Here we demonstrate a flexible, electronic device that non-invasively maps pressure-induced tissue damage, even when such damage cannot be visually observed. Using impedance spectroscopy across flexible electrode arrays in vivo on a rat model, we find that impedance is robustly correlated with tissue health across multiple animals and wound types. Our results demonstrate the feasibility of an automated, non-invasive ‘smart bandage’ for early detection of pressure ulcers. Chronic skin wounds have been called ‘a silent epidemic’ posing a significant threat to public health and the economy [1] . Each year, an estimated US$25 billion is spent on the treatment of chronic wounds [1] . They are more common in patients who are diabetic, obese or elderly; thus, the sharp increase in obesity and diabetes worldwide and the aging population in the United States—combined with the ever-increasing cost of health care—underscore the need for advances in wound care. Pressure ulcers are chronic wounds with a particularly high rate of morbidity, affecting over 2.5 million patients and costing an estimated $11 billion per year in the United States alone [1] . A pressure ulcer develops when pressure is applied to a localized area of the body over a period of time, such as when a patient lies in the same position during a lengthy surgery, stays in the ICU or has limited mobility. Injury typically occurs over a bony prominence, such as the sacrum, heels or the back of the skull [1] , [2] , [3] , [4] . The pressure causes a loss of blood flow to the tissue resulting in necrosis, and subsequent infection is a major concern. The combination of pressure, time and ischaemia-reperfusion cycles that results in a pressure ulcer varies widely between patients [1] , [2] , [3] , [4] , making them difficult to predict. Damage can occur from an ischaemic event as short as 2 h [2] , [3] , [4] , and the initial stages of damage are not easily detectable with the naked eye. By the time a surface wound is visible, the underlying tissue damage is often severe [2] , [3] , [4] . Prevention of pressure ulcers currently relies on labour-intensive vigilance in nursing care [3] , [4] , [5] . Patients are manually turned nearly every hour to relieve pressure, and high-risk areas are visually inspected for pressure ulcers [3] . Pressure-sensitive devices can alert nursing staff when a threshold of pressure is exceeded. However, it is the progressive tissue damage that determines ulcer development, not the instantaneous pressure itself. Accurate correlations between the amount of pressure, duration of pressure and ulcer development across patient populations do not exist. In effect, no clinically relevant method exists to detect progressive tissue damage to indicate whether a patient is at imminent risk of developing an ulcer. A body of literature exists that has both measured and modelled the electrical changes in cells and tissue both in vivo and in vitro , as well as provided correlations between electrical properties and cell types; this work has been summarized previously [6] , [7] , [8] , [9] , [10] , [11] . From an electrical perspective, a cell can be represented as an ion-rich conductive centre (cytoplasm) embedded in an ion-rich conductive medium (extracellular fluid), separated by a relatively non-conductive barrier (cell membrane). These ion-rich media can be described in terms of their ability to conduct charge by modelling them as resistances. Likewise, barriers to charge flow (for example, the cell membrane) can be modelled as electrical capacitances. The combination of the loss terms (that is, resistance) and energy storing terms (that is, capacitance and inductance) is known as electrical impedance. Because the impedance of a material is a function of the electrical signal being passed through it, impedances are measured across many frequencies to form a spectrum plot, which is known as impedance spectroscopy. The complex impedance Z of a medium can be expressed in polar form as with magnitude |Z| and phase angle θ , or in Cartesian form as with resistance R and reactance X . The reactance X represents the energy storage term; from equations (1) and (2), we see that a material with a higher capacity for energy storage (or polarization) will exhibit a larger reactance, X , and a larger phase angle, θ . Certain disturbances of the biological structures result in detectable changes in the impedance spectrum. For example, in vitro impedance measurements have been shown to detect cell proliferation and cell–drug interaction [12] , quantify biomass in suspensions [11] , [13] and create two-dimensional images of cell migration [14] . Much of this work utilizes the electrical ‘signature’ of the cell membrane: a well-functioning cell membrane is relatively impermeable and thus behaves like a capacitor in the presence of electric current [9] , [10] , [11] , [13] , [15] . Cell damage or death results in a loss of membrane structure and integrity, allowing ions and current to pass through the membrane. Thus, damaged cells will exhibit higher electrical conductance through the membrane and less capacity to store charge [10] ; in other words, the cell behaves less like a capacitor and more like a resistor. In an impedance measurement, this manifests itself as a phase angle θ closer to zero (or equivalently, a smaller reactance, X ). Impedance measurements of tissues in vivo have also correlated better tissue health with more reactive impedance values: bioelectrical impedance analysis of patients at high risk for developing pressure sores (as determined by the Braden scale [16] ) exhibited lower reactance and phase angle than the control group [17] . Further studies have observed that reactance increases with epidermal proliferation and granulation, and decreases with infection and cell loss, suggesting that a larger phase angle indicates healthier cell membranes while a decreased phase angle indicates impaired membrane function [18] . Many researchers are actively exploring this area; in fact, clinical trials [19] are underway and impedance-based wound monitoring devices have been patented [20] . These results led us to hypothesize that pressure ulcers may be able to be detected and diagnosed based on the changes in electrical impedance caused by the loss of cellular integrity or cell death following an ischaemia/reperfusion event. Here we report a flexible, electronic device that non-invasively detects pressure-induced tissue damage, even when such damage cannot be visually observed. Using impedance spectroscopy across flexible electrode arrays in vivo on a rat model, we find that the frequency spectra of impedance measurements are correlated in a robust way with the state of the underlying tissue across multiple animals and wound types. Flexible and stretchable electronics for biomonitoring applications is currently an area of intense research focus [21] , [22] , [23] , [24] ; our results demonstrate the feasibility of an automated, non-invasive ‘smart bandage’ for early diagnosis of pressure ulcers, improving patient care and outcomes. Multiplexed electrode array maps tissue impedance We have designed and implemented an electronic sensing device that measures spatially correlated complex impedance in vivo using a multiplexed electrode array. The device consists of an electrode array to contact the skin and control hardware that performs impedance spectroscopy across the array. The following two versions of the electrode array were developed: (1) a commercial rigid printed circuit board with gold-plated electrodes, and (2) a flexible bandage-like array produced using inkjet printing on a plastic substrate. The rigid device was a robust calibration platform that allowed us to develop the method of detecting pressure ulcers using impedance spectroscopy while, in parallel, developing the flexible device to use that method in vivo . Notably, the rigid array and the flexible array provided similar results ( Fig. 1 ), and both types were used in our experiments to collect impedance data. 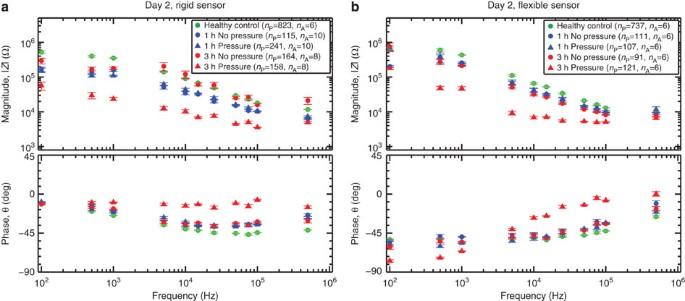Figure 1: Average impedance using rigid versus flexible array. Impedance spectra for ‘pressure’ and ‘no pressure’ locations of reversible (1 h) and irreversible (3 h) pressure damage, comparing results from the rigid (a) versus flexible (b) sensor array. Impedance data includes all animals in the study measured day 2. Markers indicate the average data values at each frequency, with error bars showing the s.e.m..nPelectrode pairs were used the calculation of the average values, measured from wounds onnAanimals. A detailed comparison of the specifications of the rigid and flexible arrays is given in Supplementary Table 1 . The rigid array was a custom printed circuit board purchased from Advanced Circuits (three layer FR4, 1 oz. copper on all layers, 1.5 mm overall thickness). The fabrication process of the printed array is illustrated in Fig. 2a,b . Gold nanoparticle ink was inkjet printed on a thin (35 μm) polyethylene naphthalate substrate. Such thin substrates enhance conformity of the printed array, improving electrode–skin contact. A sintering step was required to fuse together gold nanoparticles in the ink to create conductive lines [25] . These conductive lines were encapsulated by spin coating an amorphous fluoropolymer (Cytop); vias over the electrodes were then selectively opened using oxygen plasma etching with a shadow mask. Since several replicate printed arrays were used during animal experiments, minimizing processing variability was essential. The fabrication process proved highly reproducible: for five different arrays we observed low batch-to-batch variation in electrical properties ( Supplementary Fig. 1 ). For the five arrays, s.d. of the mean sheet resistance was extremely low, σ μ, Rs =0.01 Ω/ sq . Printed features demonstrated conductivity of 8.0 × 10 4 S cm −1 (20% of the bulk conductivity of gold), which is comparable to reported conductivity values in the literature [26] . Mechanical stability of the printed lines was another key concern because the sensor array needed to survive the wear and tear experienced during data collection. Since the arrays were subjected to both bending and torsion, we tested mechanical robustness by torsionally loading an array with angle of twist, ϕ =30°. Even after 1,000 cycles, we did not observe significant alteration of the printed structures ( Fig. 2d ). Figure 1: Average impedance using rigid versus flexible array. Impedance spectra for ‘pressure’ and ‘no pressure’ locations of reversible (1 h) and irreversible (3 h) pressure damage, comparing results from the rigid ( a ) versus flexible ( b ) sensor array. Impedance data includes all animals in the study measured day 2. Markers indicate the average data values at each frequency, with error bars showing the s.e.m.. n P electrode pairs were used the calculation of the average values, measured from wounds on n A animals. 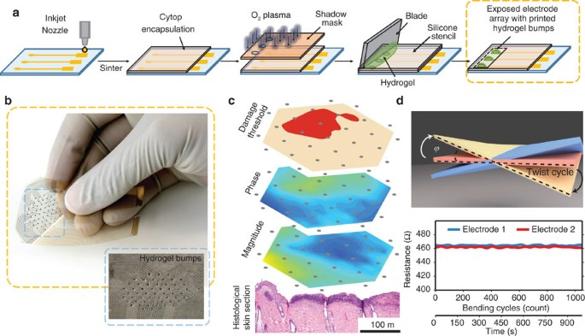Figure 2: Flexible electrode array fabrication and characterization. (a) Fabrication flow for the inkjet printed flexible electrode array. (b) An inkjet printed array, showing the hexagonal configuration of 55 equally spaced gold electrodes; inset shows printed hydrogel bumps on the fabricated array. (c) Schematic representation of the device operation. The array is placed on a woundin vivoand the electrical impedance is collected for each pair of neighbouring electrodes. A map of impedance magnitude, phase angle and damage threshold (indicated here in red) are constructed based on the location of each measurement pair. (d) Mechanical robustness testing by torsionally loading the array with angle of twistϕ=30°, with no significant change in line resistance after 1,000 twist cycles. Full size image Figure 2: Flexible electrode array fabrication and characterization. ( a ) Fabrication flow for the inkjet printed flexible electrode array. ( b ) An inkjet printed array, showing the hexagonal configuration of 55 equally spaced gold electrodes; inset shows printed hydrogel bumps on the fabricated array. ( c ) Schematic representation of the device operation. The array is placed on a wound in vivo and the electrical impedance is collected for each pair of neighbouring electrodes. A map of impedance magnitude, phase angle and damage threshold (indicated here in red) are constructed based on the location of each measurement pair. ( d ) Mechanical robustness testing by torsionally loading the array with angle of twist ϕ =30°, with no significant change in line resistance after 1,000 twist cycles. Full size image Before the sensing array was placed onto the skin, a thin layer of highly conductive hydrogel was selectively printed onto the electrodes using a silicone stencil; Supplementary Fig. 2 illustrates the attachment of the sensor array to the wound. The hydrogel was used on both the rigid and flex arrays to reduce the contact impedance between the electrode and the tissue sample being measured, improving the reliability of the measurements [27] . During operation, the array control hardware selects two electrodes in the array and performs an impedance measurement across these electrodes using a precision LCR meter; by cycling through pairs, all of the nearest neighbours of the array can be sampled and a map of the impedance measurements can be constructed ( Fig. 2c ). ‘Four-point’ measurements were also performed but were found to be much harder to correlate to wound state (see discussion in the Supplementary Information ). Registration marks were stained onto the skin to establish the position of the electrodes with respect to the pressure ulcer being measured. Impedance spectrum correlates to tissue health To create pressure ulcers, rats were sedated and the dorsal body hair was shaved and depilated with Nair to provide bare skin for impedance measurements. After the area was cleaned, the skin was gently tented up and placed between two disc-shaped magnets [28] . The animals returned to normal activity with the magnets in place for 1 or 3 h, at which point they were sedated and the magnets were removed. Eleven of the 12 animals used in this study received the 1-h treatment, and nine of the 12 animals received the 3-h treatment. Using fluorescence angiography to image real-time blood flow in the tissue ( Supplementary Information and Supplementary Fig. 3 ), we observed that relieving the pressure initially resulted in increased perfusion (reactive hyperaemia) [4] , [29] as the blood returned to the affected tissue. When blood returns to the ischaemic tissue, it produces reactive oxygen species and free radicals that can accelerate cell death [30] , [31] . In our model, 1 h of pressure produced mild reversible tissue damage, and 3 h of pressure produced more severe irreversible damage. Following the ischaemic event, we tracked the wounds for at least 3 days using impedance spectroscopy. The system measured impedance using a 100-mV RMS constant voltage test signal at frequencies between 10 2 and 10 6 Hz across all nearest-neighbour electrode pairs on the array; data from a single representative wound in the 3-h ischaemia group is shown in Fig. 3 . Across all animals in the 3-h group ( n =9), the impedance spectra for areas developing pressure ulcers were clearly distinguishable by day 3 (or earlier) from spectra for areas that were healthy. Qualitatively, wounded areas showed a decrease in impedance magnitude and phase angles closer to zero. The tissue appeared less capacitive and more conductive, consistent with a loss of cell membrane integrity [10] ( Fig. 3a ). In the impedance spectra ( Fig. 3b ), we observed that the dominant pole for the wounded tissue was at a lower frequency than for the healthy tissue. To determine specific threshold values of impedance magnitude and phase that defined ‘damaged tissue’, we utilized impedance spectra collected with the flexible electrode array from 14 wounds on eight rats. We then used a contrast optimization process that identified 15 kHz as the frequency at which the maximum difference was observed in impedance between damaged and non-damaged tissue. We determined that a magnitude value of | Z |=6 kΩ and a phase window of −30°≤ θ ≤−10° measured at 15 kHz was an effective threshold for identifying damaged tissue while avoiding false-positive readings. (See Methods section for a discussion of the damage threshold values used for impedance measured with the rigid calibration array.) The same threshold values were applied to all wounds, regardless of whether they belonged to the 1-h or 3-h treatment group. Any pair of electrodes whose magnitude was below the threshold and whose phase value fell within the specified window was labelled as ‘damaged tissue’. In other words, the term ‘damage’ indicates regions where impedance data predicts tissue damage, whereas the term ‘pressure’ indicates data from any area of tissue subjected to magnet pressure. The phase requirement was included to make the damage parameter less susceptible to minor animal-to-animal skin variations than using magnitude alone (such as skin thickness, hydration status and so on), and thus improve the reliability of tissue classification. Spatial impedance data can thus be translated into a map of the tissue damage parameter that differentiates healthy tissue from a wound. As shown in Fig. 3 , by day 2 (the day following the ischaemic event) the impedance sensor identified an area of tissue damage that correlates with the placement of the magnets. Not surprisingly, tissue damage within the pressure area is not uniform; an ulcer can be seen in the lower right region of the pressure area in the day 3 image in Fig. 3a , and this region is also highlighted in the map of the damage threshold. The analysis shown in Fig. 3a,b was carried out for each wound on each animal in the study, and all animals in the 3-h treatment group produced similar results. The repeatability of the results across wounds on many animals is shown in Fig. 3c . Here the impedance spectra for reversible (1 h) and irreversible (3 h) pressure damage measured with the flexible array on day 2 were averaged over all animals in the study, excluding those killed before day 2. For each wound, each electrode pair was labelled either as ‘pressure’ or ‘no pressure’ depending on whether or not the electrodes measured tissue where pressure had been applied. (All pairs spanning the boundary of ‘pressure/no pressure’ were omitted.) The reduction in impedance magnitude and a phase angle closer to zero is clearly evident in this ensemble data for the 3-h pressure group. 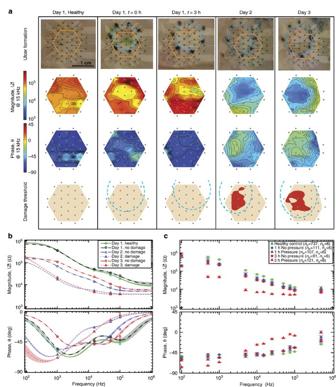Figure 3: Impedance spectrum correlates to tissue damage. (a) The progression of a representative example of irreversible tissue damage created with a 3-h ischaemia cycle is shown on days 1–3. On day 1, healthy is a control measurement taken before ulcer formation,t=0 h corresponds to measurements immediately following magnet removal, andt=3 h corresponds to measurements after 3 h of reperfusion. Row 1: the transparent, flexible electrode array is in place over the wound, and the pressure area is indicated with a dashed blue circle. The outer ring of electrodes on the array was not used for the two-point impedance measurements shown here; the hexagon overlaid on the image outlines the area corresponding to the impedance maps. Scale bar (1 cm) applies to all wound photos. Rows 2 and 3: impedance magnitude and phase angle measured across nearest-neighbour pairs with the flexible electrode array at a frequency of 15 kHz. The asymmetry in the surface map on day 3 is due to the rejection of one broken electrode (see Methods section). Row 4: the damage threshold is determined from the magnitude and phase data at each pair, and mapped across the array. Red indicates tissue damage. On days 2 and 3, a region of tissue damage is detected that clearly correlates with the location of the developing pressure ulcer. (b) Impedance spectra for the wound shown inaof healthy skin before applying pressure, ‘No damage’ regions on days 1–3, and ‘Damage’ regions on days 2 and 3. A representative electrode pair was selected from each region. The markers indicate the measured data values, whereas the lines and the shaded regions indicate the estimated transfer function and the 95% fit confidence interval, respectively. (c) Impedance spectra for ‘pressure’ and ‘no pressure’ locations of reversible (1 h) and irreversible (3 h) pressure damage measured with the flexible array on day 2, averaged over all animals in the study. Markers indicate the average data values at each frequency, with error bars showing the s.e.m..nPelectrode pairs went into the calculation of the average values, measured from wounds onnAanimals. Figure 3: Impedance spectrum correlates to tissue damage. ( a ) The progression of a representative example of irreversible tissue damage created with a 3-h ischaemia cycle is shown on days 1–3. On day 1, healthy is a control measurement taken before ulcer formation, t =0 h corresponds to measurements immediately following magnet removal, and t =3 h corresponds to measurements after 3 h of reperfusion. Row 1: the transparent, flexible electrode array is in place over the wound, and the pressure area is indicated with a dashed blue circle. The outer ring of electrodes on the array was not used for the two-point impedance measurements shown here; the hexagon overlaid on the image outlines the area corresponding to the impedance maps. Scale bar (1 cm) applies to all wound photos. Rows 2 and 3: impedance magnitude and phase angle measured across nearest-neighbour pairs with the flexible electrode array at a frequency of 15 kHz. The asymmetry in the surface map on day 3 is due to the rejection of one broken electrode (see Methods section). Row 4: the damage threshold is determined from the magnitude and phase data at each pair, and mapped across the array. Red indicates tissue damage. On days 2 and 3, a region of tissue damage is detected that clearly correlates with the location of the developing pressure ulcer. ( b ) Impedance spectra for the wound shown in a of healthy skin before applying pressure, ‘No damage’ regions on days 1–3, and ‘Damage’ regions on days 2 and 3. A representative electrode pair was selected from each region. The markers indicate the measured data values, whereas the lines and the shaded regions indicate the estimated transfer function and the 95% fit confidence interval, respectively. ( c ) Impedance spectra for ‘pressure’ and ‘no pressure’ locations of reversible (1 h) and irreversible (3 h) pressure damage measured with the flexible array on day 2, averaged over all animals in the study. Markers indicate the average data values at each frequency, with error bars showing the s.e.m.. n P electrode pairs went into the calculation of the average values, measured from wounds on n A animals. Full size image Impedance spectroscopy identifies damage that is not visible The ability to detect and monitor a pressure ulcer that has already formed on a patient is valuable, but a key advantage of using impedance spectroscopy to detect pressure ulcers is early detection of tissue damage. Mild, reversible pressure damage was created using a 1-h ischaemia cycle (as opposed to the 3-h ischaemia cycle used above), then monitored with impedance measurements for 3 days. The skin appeared slightly white during reperfusion, but no visible ulcer developed in the following 9 days, indicating that any pressure-induced damage was truly reversible. The impedance measurements reveal a more nuanced story. Using the same impedance thresholds to detect damage that were used for irreversible damage, we found that the impedance sensor detected damaged tissue in the region of pressure application in just over half of the cases studied (6 out of 11 animals using the rigid array and 5 out of 7 animals using the flexible array), again with no false-positive results ( Fig. 4 ). Owing to the expected animal-to-animal variation, we hypothesize that the combination of pressure and duration used in the 1-h cases was sufficient to create tissue damage in some, but not all, animals. Histology of skin samples with 1 h of ischaemia confirmed that the tissue was not damaged in all cases. Variation in damage severity was also observed in 3 h ischaemia cases, with some ulcers reaching a stage II classification while others with the same treatment were only classified as a stage I ulcer [3] . This animal-to-animal variation observed for the 1-h pressure cases (as well as the non-uniform damage within the area of pressure application) explains why averaging the impedance of ‘pressure’ and ‘no pressure’ areas over many animals ( Fig. 3c ) obscures a meaningful result for the reversible damage case. We observed the following three outcomes in response to applied pressure ( Fig. 5 ): (1) severe, irreversible pressure damage is sustained creating a visible ulcer that is also detected with impedance spectroscopy ( Fig. 5a ); (2) mild pressure damage is sustained that is not visible to the naked eye, but can be detected using impedance spectroscopy ( Fig. 5b ); and (3) pressure is not sufficient to damage the tissue and, correspondingly, the impedance sensor does not indicate damage ( Fig. 5c ). Figure 5 also demonstrates that the rigid calibration and flexible printed sensor arrays produced similar results, but that the rigid arrays produced more complete damage maps because they were more robust during multiple measurement–disinfection cycles (see Methods section). 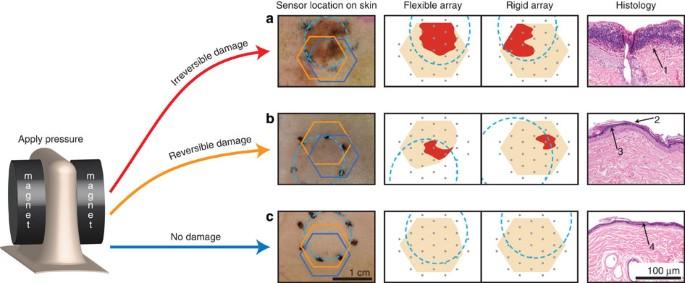Figure 5: Early detection of pressure-induced tissue damage. Magnets were used to create a pressure ulcer model on ratsin vivo. We observed the following three outcomes influenced by the amount of pressure, the duration of treatment and animal-to-animal variation: irreversible damage was detected both visually and electrically; (a) reversible damage was detected electrically but not visually; (b) and no damage was detected visually or electrically (c). Histological analysis indicated loss of epidermis (1) and ulceration when there was irreversible tissue damage, hyperkeratosis (2) and hypergranulosis (3) when the damage was measurable but reversible, and focal hyperkeratosis (4) in the scenario where no damage is detected. Representative wound images with sensor locations indicated, damage parameter maps obtained from those wounds using flexible and rigid sensor arrays, and histology results are shown for each scenario. Dashed light blue circles indicate where the pressure was applied to the skin, orange and dark blue hexagons indicate the location of the flexible and rigid arrays on the wound, respectively, and grey dots represent the electrodes. Scale bars, 1 cm (for wound photos) and 100 μm (for histology images). 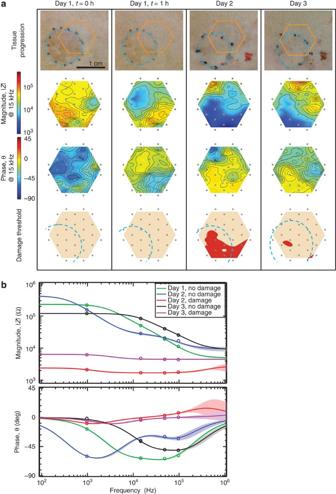The second observation—detecting changes in the tissue that cannot be seen by eye—demonstrates the sensitivity of impedance spectroscopy to physiological changes associated with ulcers and its applicability as an early detection method for pressure ulcers. Figure 4: Impedance maps identify mild, reversible pressure damage. (a) The progression of reversible pressure damage created with a 1-h ischaemia cycle is shown on days 1–3. Dashed grey circles indicate where the pressure was applied and dots represent the placement of the electrodes. Slight discolouration of the skin is observed immediately after removing the magnets, but no ulcer develops. Impedance magnitude and phase were measured with the rigid printed circuit board array. Damage is detected electrically on day 2 even with no visible evidence of the pressure damage, demonstrating the early detection capability of the device. (The small abrasion to the right of the measured area was irritation from hair removal.) Only a small region of damage remains on day 3. Scale bar (1 cm) applies to all wound photos. (b) A Bode diagram showing the impedance magnitude and phase versus frequency of ‘No damage’ and ‘Damage’ regions on days 1–3. A representative electrode pair was selected from each region. The circle markers indicate the measured data values, whereas the lines and the shaded regions indicate the estimated transfer function and the 95% fit confidence interval, respectively. Figure 4: Impedance maps identify mild, reversible pressure damage. ( a ) The progression of reversible pressure damage created with a 1-h ischaemia cycle is shown on days 1–3. Dashed grey circles indicate where the pressure was applied and dots represent the placement of the electrodes. Slight discolouration of the skin is observed immediately after removing the magnets, but no ulcer develops. Impedance magnitude and phase were measured with the rigid printed circuit board array. Damage is detected electrically on day 2 even with no visible evidence of the pressure damage, demonstrating the early detection capability of the device. (The small abrasion to the right of the measured area was irritation from hair removal.) Only a small region of damage remains on day 3. Scale bar (1 cm) applies to all wound photos. ( b ) A Bode diagram showing the impedance magnitude and phase versus frequency of ‘No damage’ and ‘Damage’ regions on days 1–3. A representative electrode pair was selected from each region. The circle markers indicate the measured data values, whereas the lines and the shaded regions indicate the estimated transfer function and the 95% fit confidence interval, respectively. Full size image Figure 5: Early detection of pressure-induced tissue damage. Magnets were used to create a pressure ulcer model on rats in vivo . We observed the following three outcomes influenced by the amount of pressure, the duration of treatment and animal-to-animal variation: irreversible damage was detected both visually and electrically; ( a ) reversible damage was detected electrically but not visually; ( b ) and no damage was detected visually or electrically ( c ). Histological analysis indicated loss of epidermis (1) and ulceration when there was irreversible tissue damage, hyperkeratosis (2) and hypergranulosis (3) when the damage was measurable but reversible, and focal hyperkeratosis (4) in the scenario where no damage is detected. Representative wound images with sensor locations indicated, damage parameter maps obtained from those wounds using flexible and rigid sensor arrays, and histology results are shown for each scenario. Dashed light blue circles indicate where the pressure was applied to the skin, orange and dark blue hexagons indicate the location of the flexible and rigid arrays on the wound, respectively, and grey dots represent the electrodes. Scale bars, 1 cm (for wound photos) and 100 μm (for histology images). Full size image Cell membrane disruption correlates with impedance change Histological cross-sections performed at various time points throughout the study ( Figs 5 and 6 ) support the hypothesis that the alteration of cell membranes and tissue structure causes the observed impedance changes. Histological analysis was performed on tissue samples from reversible (1 h of ischaemia) and irreversible (3 h of ischaemia) pressure groups. Histopathological examination of the haematoxylin and eosin-stained sections showed focal compact hyperkeratosis and focal hypergranulosis in the area of magnet application in both 1 and 3 h groups. The skin samples from the 1-h application group showed no evidence of skin ulceration, while all samples taken after the 3-h magnet application period demonstrated ulceration. These lesions showed overlying necroinflammatory debris with serum crust, focal loss of epidermis, alteration of underlying collagen and had sparse to moderate amounts of mixed inflammatory infiltrate composed predominantly of lymphocytes and neutrophils. In some cases, the inflammatory infiltrate involved deeper dermis, skeletal muscle and fascia. These histological findings were consistent with the changes in tissue structure that are expected to cause changes in impedance [10] . 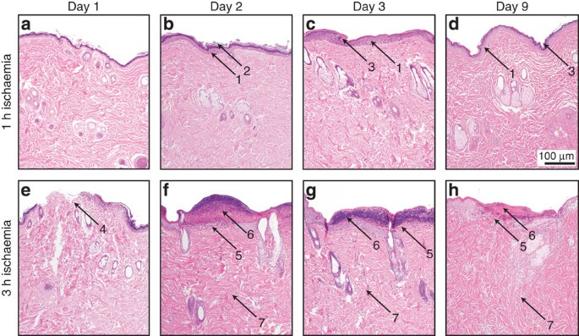Figure 6: Histology of skin samples. Skin samples were collected for histology on days 1, 2, 3 and 9, and processed with haematoxylin and eosin staining. Samplesa–dwere taken from animals in the 1-h pressure treatment group, whereas samplese–hwere taken from animals in the 3-h pressure treatment group. All images were taken with × 100 magnification. (a) Normal-looking dermis and epidermis. (b) No signs of ulceration. Normal epidermis (1) with orthokeratosis (2). (c,d) No signs of ulceration. Normal epidermis (1) with compact hyperkeratosis (3). (e) Early small ulcer (4). (f–h) Loss of epidermis (5) and necroinflammatory debris (scab, 6) with inflammation (neutrophils and lymphocytes, 7) deeper in the dermis. Scale bar (100 μm) applies to all images. Figure 6: Histology of skin samples. Skin samples were collected for histology on days 1, 2, 3 and 9, and processed with haematoxylin and eosin staining. Samples a – d were taken from animals in the 1-h pressure treatment group, whereas samples e – h were taken from animals in the 3-h pressure treatment group. All images were taken with × 100 magnification. ( a ) Normal-looking dermis and epidermis. ( b ) No signs of ulceration. Normal epidermis (1) with orthokeratosis (2). ( c , d ) No signs of ulceration. Normal epidermis (1) with compact hyperkeratosis (3). ( e ) Early small ulcer (4). ( f – h ) Loss of epidermis (5) and necroinflammatory debris (scab, 6) with inflammation (neutrophils and lymphocytes, 7) deeper in the dermis. Scale bar (100 μm) applies to all images. Full size image Applications extend beyond pressure ulcers In addition to the detection of pressure ulcers, we have also demonstrated that our device can track the state of open skin wounds ( Supplementary Information and Supplementary Fig. 4 ). Our measurements confirm that we can identify not only the size and shape of an excision by determining the border of the wound but we can also differentiate between a moist wound (exposed wound bed, potentially pus and so on) and a healing, scab-covered wound. With a slight change in instrumentation, the same device can also be used to measure voltage at each electrode with respect to a common reference, creating a map of the voltage and endogenous electric field across the wound. It is well known that cells can be directed to migrate with an applied electric field [32] , [33] , [34] , [35] , [36] , and there is evidence, although somewhat controversial, that applying an electric field may assist in the healing process [37] . The device demonstrated here provides the capability to test the extension of these theories from cells to complex tissues in vivo . Thus, it could be adapted to sense the endogenous field, apply an external field and monitor the response of the tissue to the stimulus, providing much-needed evidence regarding the efficacy of electrical stimulation for healing chronic wounds. We have developed a non-invasive electrical sensing device that utilizes impedance spectroscopy to detect pressure-induced tissue damage in a rat model in vivo . The sensitivity of this detection method and the robustness of the calculated damage parameter are sufficient to detect mild, reversible physiological changes that are not apparent by visual inspection. While the specific threshold values that indicated tissue damage in this study demonstrate the capability of impedance spectroscopy as a technique for early detection of tissue wounds, additional studies will be needed to determine clinically relevant threshold values in human patients. A commercial device with this capability could have a marked impact on the standard of care for pressure ulcers. Disease prevention is a well-recognized approach in medicine; providing an early detection mechanism for pressure damage would allow caregivers to respond proactively, preventing any further damage to the tissue and enabling close monitoring of tissue condition. Further, the variation in wound severity that we observed for a given treatment (which is not unique to our model) strongly supports the value of a device that directly measures the status of the tissue, rather than relying on secondary measurements such as applied pressure. If the subtle changes in tissue are detected early enough, as demonstrated here in the case of the reversible 1 h pressure damage, the formation of pressure ulcers in some patients may be prevented entirely, greatly reducing health-care costs and improving patient outcomes. Inkjet printed electrode array The flexible sensor array was inkjet printed on top of planarized polyethylene naphthalate substrates (DuPont). Harima gold nanopaste ink (model: NPG-J) was printed with 30 μm drop spacing using a Dimatix Materials Printer (DMP-2800). Printed features were cured with a slow ramp annealing step (30–230 °C with 0.7 °C per min ramp), followed by a constant temperature bake at 230 °C for 60 min. Thickness of the printed lines ranged from 0.5 to 1 μm. An amorphous fluoropolymer (Cytop CTX-809 A) coating was then spun at 1,200 r.p.m. for a 100-nm film thickness. Electrode vias were opened using oxygen plasma etching. Electrical sheet resistance measurements were measured using four-point probe measurements. Various layer thicknesses of the sensor were measured with a Dektak Profilometer. Rat model for pressure ulcers Wild-type rats (Sprague–Dawley, 250–300 g, 8 weeks old, male) were anaesthetized with isofluorane mixed with oxygen. Hair was shaved from the back, depilated with Nair and then the area was cleaned with mild detergent (Dawn) and isopropyl alcohol. The skin was gently tented up and placed between two round, flat magnets (5 × 12 mm diameter, 2.4 g weight and 1,000 G magnetic force). This procedure left a 5-mm skin bridge between the magnets, creating ~50 mm Hg pressure between the plates. Rats tolerated the procedure well, returning to normal activity within a few minutes with the magnets in place. Magnets were removed after 1 or 3 h, and impedance measurements were taken while rats were under isofluorane anaesthesia daily for 3 days. Rats received a 1-h treatment and a 3-h treatment on different areas of the back on separate days; the animals killed for histological analysis on the day of pressure treatment received either the 1- or 3-h treatment but not both. Study sample size was chosen in consultation with a professional statistician at University of California, San Francisco to minimize animal numbers and suffering while providing statistically significant results. All procedures were reviewed and approved by the University of California San Francisco Institutional Animal Care and Use Committee (approval number AN100403-01C). Skin samples for histology Full thickness skin wounds were excised, immediately placed flat in cassettes and stored in 10% neutral-buffered formalin for 24–72 h. Tissue was then transferred to 70% ethanol and stored for up to 1 week. Samples were embedded in paraffin and sectioned at 5 microns. Slides were stained with haematoxylin and eosin. Impedance measurements Impedance magnitude and phase were measured using an Agilent E4980AL 20 Hz to 1 MHz Precision LCR meter with a 100-mV constant voltage sine wave output signal with a frequency of 100 Hz to 1 MHz. Each electrode on the array can be independently selected by the control hardware, allowing pairwise impedance measurements between electrodes. Custom software implemented in Python communicated with the control hardware to select electrode pairs in a specified sequence, and simultaneously controlled the LCR meter. A microcontroller on the control board routed the test signal from the LCR meter to the selected electrodes, the impedance was recorded and then the microcontroller selected the next set of electrodes in the measurement sequence. Impedance data were analysed using a suite of custom MATLAB scripts utilizing the Statistics, System Identification and Control System Toolboxes. Contact impedance and stray capacitance . Minimizing the effects of contact impedance and stray capacitance is critical to obtaining accurate measurements of tissue impedance. Thus, we optimized our manufacturing process to minimize contact impedance by selectively applying high-conductance gel to each electrode. This process was controlled using a patterned stencil and blade-coating method. Sufficient pressure was applied during the measurement to ensure the measurement array stayed in contact with the tissue. In addition, stray capacitance and other measurement parasitics were minimized by choosing minimum-length shielded cables to the LCR meter, properly shielded BNC (Bayonet Neill-Councelman) connections, and noise-minimizing layout and routing techniques in our custom-built control hardware. We found the Agilent Impedance Measurement Handbook to be a valuable reference in this regard (available from Agilent Technologies at http://cp.literature.agilent.com/litweb/pdf/5950-3000.pdf ). Mounting the sensor array to the wound . The procedure for mounting the sensing array on wounds is shown in Supplementary Fig. 2 . A thin polydimethylsiloxane stencil is first aligned and placed on the flexible array board to allow for selective application of hydrogel (SignaGel Electrode Gel, Parker Laboratories Inc.) to each electrode of the array. The hydrogel ensures adequate electrical contact between each electrode and the skin of the rat. After the stencil is removed, the array is placed carefully on the area of the rat’s back to be measured and secured in place with a transparent Tegaderm dressing. Finally, a piece of Coban self-adherent wrap is placed around the body of the rat to apply even pressure to the array against the rat’s skin. This mounting procedure allows the board to move with the rat’s breathing but ensures that it does not shift during measurements. The rigid array board is mounted to the rat in a similar manner. Damage threshold: flex versus rigid array . Owing to the differences in materials and assembly of the inkjet printed flexible electrode array versus the rigid calibration array ( Supplementary Table 1 ), the threshold for detecting damaged tissue was adjusted depending on which electrode array was used to record impedance data. Qualitatively, the flexible arrays had a slightly higher line resistance and an additional capacitive contribution from one extra connector between the flexible array and the control hardware, both of which need to be accounted for. Threshold values indicating tissue damage were determined separately for the flexible and rigid arrays: Flexible electrode array: | Z |≤6 kΩ and −35° ≤θ ≤−10° Rigid calibration array: | Z |≤5 kΩ and −5° ≤θ ≤10° Note that the same threshold values were used to detect damage for all wounds on all animals, regardless of wound severity (1 or 3 h pressure group). Rejecting data from damaged electrode arrays . Repeated use of the flex arrays, including the cleaning and sanitation required between each measurement, eventually resulted in damage to the printed gold lines or the encapsulation layer. The condition of the flexible arrays was tested periodically (at least twice daily, before and after wound measurements) by submerging the array in a saltwater solution (100 g l −1 NaCl) and measuring the impedance between each pair. If the impedance magnitude between any two electrodes was <100 Ω, the pair was considered ‘shorted’, and a magnitude >50 kΩ (roughly twice the expected value of the saltwater) was considered ‘open’. All analysis of impedance data measured with a flexible array was first filtered to remove any data points from electrode pairs that failed the saltwater test. As seen in Fig. 3 (day 3, right column) and Fig. 5 (reversible damage and flexible array), missing electrodes caused asymmetrical impedance maps but did not compromise the validity of the data. How to cite this article: Swisher, S. L. et al . Impedance sensing device enables early detection of pressure ulcers in vivo . Nat. Commun . 6:6575 doi: 10.1038/ncomms7575 (2015).